Deactivation of carbon electrode for elimination of carbon dioxide evolution from rechargeable lithium–oxygen cells Carbon has unfaired advantages in material properties to be used as electrodes. It offers a low cost, light weight cathode that minimizes the loss in specific energy of lithium–oxygen batteries as well. To date, however, carbon dioxide evolution has been an unavoidable event during the operation of non-aqueous lithium–oxygen batteries with carbon electrodes, due to the reactivity of carbon against self-decomposition and catalytic decomposition of electrolyte. Here we report a simple but potent approach to eliminate carbon dioxide evolution by using an ionic solvate of dimethoxyethane and lithium nitrate. We show that the solvate leads to deactivation of the carbon against parasitic reactions by electrochemical doping of nitrogen into carbon. This work demonstrates that one could take full advantage of carbon by mitigating the undesired activity. Lithium–oxygen (Li–O 2 ) batteries offer ultra-high energy storage that possibly eliminates the range anxiety of electric vehicles if realized [1] , [2] , [3] , [4] . For last several years, extensive studies on the Li–O 2 batteries with non-aqueous electrolytes have been performed by several research groups [1] , [3] , [5] , [6] , [7] , [8] . This allows us to understand the fundamentals of Li–O 2 chemistry and to identify the challenges facing for the successful operation of the Li–O 2 cells. To identify materials (in particular, electrolyte and cathode) that are stable against parasitic reactions involved with active species in the cells (intermediates such as superoxides, discharge product such as Li 2 O 2 ) is a paramount challenge. The formation and decomposition of byproducts originating other than net electrochemical reaction of Li-O 2 cells, 2(Li + +e − )+O 2 ↔Li 2 O 2 (U 0 =2.96 V versus Li/Li + ), lead to catastrophic degradation of the cells, resulting in poor rechargeability [6] , [8] , [9] , [10] , [11] . The analysis of gas evolution during the operation of Li–O 2 cells has been crucial for learning the internal chemical processes [7] , [9] , [12] . In particular, the CO 2 evolution during the charge cycle provides critical clues on the oxidative decomposition of byproducts, hence has been studied extensively. To date, no Li–O 2 cell with carbon cathode has shown cycleability without CO 2 evolution, which indicates that the carbon plays a major role for the parasitic reactions [7] , [9] . This is unfortunate since the advantageous properties of carbon (such as light weight, low cost and so on), which have been beneficial to wide ranges of electrochemical cells [13] , will not be applicable to the Li–O 2 cells. Consequently, recent research effort undergoes for searching alternative materials to carbon such as nanoporous gold (Au) and titanium carbide (TiC) [7] , [14] . Although the reversible battery operation without CO 2 evolution has been demonstrated with the alternative materials, to apply them into Li–O 2 cells leads to significant trade-offs in the specific energy and cost, hence making them impractical. Carbon certainly has unfaired advantages in material properties to be used as an electrode if one could mitigate the undesired activity. In this paper, we present an effective approach to deactivate carbon electrode using an ionic solvate of dimethoxyethane (DME) and lithium nitrate (LiNO 3 ). The interaction between the ionic solvate and active sites of carbon during the discharge process of Li–O 2 cells resulted in the formation of Pyridinic structure. The deactivation of carbon electrode leads to complete elimination of CO 2 during the charge cycle, which implies the suppression of parasitic reactions associated with carbon electrode. This work enables rechargeable Li–O 2 cells without CO 2 evolution by mitigating the undesired activity of carbon electrode. Elimination of CO 2 evolution The structural details of the Li–O 2 cell used in this study are presented schematically in Fig. 1a . A carbon black (Ketjenblack, KB) is used as the cathode material (see the methods section). The amount of O 2 and CO 2 gas evolved during the charge cycle of the cell was measured using a differential electrochemical mass spectrometry (DEMS). The analytical performance of our DEMS set-up has been discussed previously [12] . The Li–O 2 cells were discharged up to the capacity of 1 mAh (200 μA and 5 h), and the consumption of O 2 was monitored by the pressure drop. During the charge cycle, the amounts and masses of gases evolved from the cell were analysed. The galvanostatic discharge and charge profiles of two Li-O 2 cells containing 0.5 M LiNO 3 -DME and 1 M LiTFSI-DME electrolytes, respectively, are presented in Fig. 1b . While the discharge profiles of the two cells are very similar, the charge behaviour of the cells are noticeably different: the cell containing 0.5 M LiNO 3 -DME shows a plateau in charge potential while the cell with 1 M LiTFSI-DME shows rapidly increasing potential with charging time throughout the entire range of charge cycle. The scanning electron microscopy (SEM) image in Fig. 1c presents the discharge products on carbon cathode of the cell containing 0.5 M LiNO 3 -DME. The well-defined toroidal nanoparticles of Li 2 O 2 having diameters of ~300–500 nm indicates that the main reaction in the cell is the Li–O 2 electrochemistry that generates Li 2 O 2 . The X-ray diffraction analysis confirms the formation of Li 2 O 2 crystals during discharge process ( Supplementary Fig. 1 ). In contrast, the cell with 1 M LiTFSI-DME electrolyte shows no clear evidence for the growth of the toroidal nanoparticles (for 1 mAh discharge), even though deposition of Li 2 O 2 is evidenced by the gas analysis during charge cycle ( Supplementary Fig. 2 ) [15] , [16] . 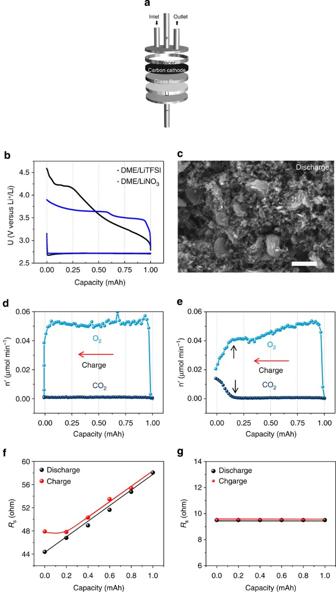Figure 1:In situDEMS, SEM and impedance measurement. (a) A schematic presentation of the Li-O2cell used in this study. (b) Galvanostatic discharge/charge profiles of the cells containing 0.5 M LiNO3-DME (blue) and 1 M LiTFSI-DME (black) electrolyte. (c) A top view SEM micrograph of the carbon cathode after 1 mAh discharge of the cell containing 0.5 M LiNO3-DME electrolyte. The scale bar indicates 500 nm. (d)In situDEMS result of the cell containing 0.5 M LiNO3-DME electrolyte. No CO2evolution is detected during the entire charging process. (e)In situDEMS result of the cell containing 1 M LiTFSI-DME electrolyte. Significant amount of CO2evolution is detected at the end of charging process. (f) The electrolyte resistance (Rs) of the cell containing 0.5 M LiNO3-DME electrolyte measured as a function of discharge and charge capacity. (g) TheRsof the cell containing 1 M LiTFSI-DME electrolyte measured as a function of discharge and charge capacity. Figure 1: In situ DEMS, SEM and impedance measurement. ( a ) A schematic presentation of the Li-O 2 cell used in this study. ( b ) Galvanostatic discharge/charge profiles of the cells containing 0.5 M LiNO 3 -DME (blue) and 1 M LiTFSI-DME (black) electrolyte. ( c ) A top view SEM micrograph of the carbon cathode after 1 mAh discharge of the cell containing 0.5 M LiNO 3 -DME electrolyte. The scale bar indicates 500 nm. ( d ) In situ DEMS result of the cell containing 0.5 M LiNO 3 -DME electrolyte. No CO 2 evolution is detected during the entire charging process. ( e ) In situ DEMS result of the cell containing 1 M LiTFSI-DME electrolyte. Significant amount of CO 2 evolution is detected at the end of charging process. ( f ) The electrolyte resistance ( R s ) of the cell containing 0.5 M LiNO 3 -DME electrolyte measured as a function of discharge and charge capacity. ( g ) The R s of the cell containing 1 M LiTFSI-DME electrolyte measured as a function of discharge and charge capacity. Full size image Figure 1d and e presents the DEMS results that render the direct comparison of the gas evolution from the two cells containing different electrolytes (that is, 0.5 M LiNO 3 -DME and 1 M LiTFSI-DME). The O 2 evolution from the cell with 0.5 M LiNO 3 -DME electrolyte increases sharply at the beginning of the charge cycle and then stays constant throughout the entire charge cycle. No CO 2 evolution was observed for this cell even at the later stage of the charge cycle. This behaviour was consistent regardless of the degree of discharge: the DEMS results of the cell discharged to the discharge cutoff potential of 2.0 V show no evidence of CO 2 evolution as well (Galvanostatic discharge/charge profiles and corresponding in situ DEMS results are shown in Supplementary Fig. 3 ). This behaviour is strikingly different from that of the cells containing other electrolytes. As shown in Fig. 1e , the DEMS result of the cell containing 1 M LiTFSI-DME shows large amount of CO 2 evolution and, coincidently, less amount of O 2 evolution during the charge cycle. It is noted that the total amount of O 2 evolved from the cell with 0.5 M LiNO 3 -DME electrolyte is ~15% more than that from the cell containing 1 M LiTFSI-DME electrolyte. To understand this unique behaviour of the Li–O 2 cell containing LiNO 3 -DME electrolyte, we carried out the impedance spectroscopy measurements at multiple points during discharge and charge cycles. Figure 1f shows the electrolyte resistance ( R s ) as a function of capacity for discharge and charge. Interestingly, the R s values of the cell with 0.5 M LiNO 3 -DME monotonically increase with increasing discharge capacity, ranging from 44.3 to 58.0 Ω. During charge cycle, the R s values decrease with charge time (which corresponds to the decrease in capacity from 1.0 mAh) until the cell potential reaches 3.7~3.8 V. The R s value shows some hysteresis at the end of charge cycle and remains ~4 Ω higher than the R s at the beginning of discharge. In contrast, the R s values for the cell containing LiTFSI-DME (shown in Fig. 1g ) stay almost constant during the discharge and charge cycles. Since the number of conductive species (dominantly salt ions) in the electrolyte determines the R s value, the changes in R s with LiNO 3 -DME indicate that the number of conductive species decreases with discharge time and reversibly increases during charge cycle. There are some degrees of irreversible changes in the number of conductive species at the end of discharge/charge cycle, which results in the hysteresis in R s value. Deactivation of carbon cathode Previously, experiments using the carbon isotope (99% 13 C) cathode have suggested that the carbon in the CO 2 gas evolved from the cells is originating from both electrolyte and cathode [9] , [12] . The complete elimination of CO 2 evolution presented in Fig. 1 , therefore, indicates that the combination of LiNO 3 salt and DME solvent plays a crucial role to interrupt the parasitic reactions that are involved with both cathode and electrolyte. To elucidate the details behind this CO 2 -evolution-free charging behaviour, we performed sets of experiments. A linear sweep voltammetry measurement was performed for the cell containing 0.5 M LiNO 3 -DME under argon (Ar) gas environment ( Supplementary Fig. 4a ). A clear oxidation peak was observed at the potential near 3.6 V, which suggests that an oxidation reaction takes place on the carbon surface. The product of this oxidation reaction was revealed by the complementary in situ DEMS results ( Supplementary Fig. 4b ), which confirms the evolution of NO gas at the potential of the oxidation peak in the linear sweep voltammetry. This indicates that the origin of the peak near 3.6 V is the oxidation of surface compound(s) containing N and O. The existence of this surface compound(s) (we call this as surface layer) on carbon cathode is further evidenced by N1s X-ray photoelectron spectroscopy (XPS) analysis ( Supplementary Fig. 4c ). The XPS data show a peak at binding energy of ~406 eV, which corresponds to NO x species [17] . It should be noted that the mixtures of glymes and lithium salts have been well known to form ionic associations (solvates), which often contain crystalline phases [18] , [19] . Among various anions, the NO 3 − forms very strong ionic association with DME [18] , [19] , [20] . The surface layer containing NO x species on the carbon is, therefore, believed to be the solvate of LiNO 3 and DME (such as contact ion pair between a DME molecule and Li + and NO 3 − ) [18] , [19] , [20] . It seems the surface layer does not affect the oxidation of Li 2 O 2 during the charging process of the Li–O 2 cells as shown by the DEMS results of a Li–O 2 cell containing 0.5 M LiNO 3 -DME electrolyte ( Supplementary Fig. 5 ). There was no NO gas evolution at the oxidation potential of the NO x species during the charging process of the Li–O 2 cell. The N1s XPS spectra of the carbon cathode after discharge process give more insights into the role of the LiNO 3 -DME solvate. The carbon cathode was pretreated with LiNO 3 -DME solvate, and 1 M LiTFSI-DME was used as the electrolyte for the Li–O 2 cell ( Supplementary Fig. 6 ). The XPS result in Fig. 2a shows a strong new peak at ~398 eV in addition to the NO x peak at ~406 eV. The characteristic peak at ~398 eV of carbon is well known as the binding energy of the N1s in Pyridinic structure [21] , [22] , [23] , [24] . The existence of the Pyridinic structure, therefore, evidences the doping of nitrogen into carbon cathode during discharge process. Further, since the carbon in contact with the solvate at the open circuit voltage only shows NO x species on the surface ( Supplementary Fig. 4 ), the formation of the Pyridinic structure is most likely driven by electrochemical process during the discharge of the cell. This also implies that the NO x species of the surface layer is used as the source of nitrogen. The nitrogen doping of carbon, which typically takes place by the interaction of N-containing molecules with oxygenated groups on carbon (such as −OOH, =O, −OH) and subsequent transformation into Pyrrolic or Pyridinic structures, leads to the loss of active sites on carbon surface [21] , [25] . The reaction between the solvate and active sites of carbon cathode in Li–O 2 cells, therefore, deactivates the carbon against parasitic reactions [26] . This is supported by the DEMS results ( Supplementary Fig. 6b ) showing less amount of CO 2 evolution when the carbon cathode is treated with the solvate. To completely eliminate the CO 2 evolution, however, the parasitic reactions involved with electrolytes should be suppressed as well. Previous work shows that the formation of carbonates (resulting from the decomposition of electrolyte solvent) is significantly hindered when inert materials, such as nanoporous Au or TiC [7] , [14] , are used as the cathode. Further, the hydrophilicity of carbon is reported to be a governing parameter for the CO 2 evolution [9] . These suggest that the carbon in the cathode is involved with the parasitic reactions to decompose the electrolytes and the surface functional groups of carbon play a critical role for the parasitic reactions. We used the carbon isotope ( 13 C) as the cathode to investigate the carbon’s role for the decomposition of electrolyte solvent using DEMS measurements. Two cells were prepared using 1 M LiTFSI-DME as an electrolyte: one has cathode of pristine 13 C and the other has 13 C pretreated with LiNO 3 -DME solution. The DEMS results evidence that the pretreated cathode evolves less amount of CO 2 originated from both electrolyte ( 12 CO 2 in Supplementary Fig. 7a ) and cathode ( 13 CO 2 in Supplementary Fig. 7b ). This is in good agreement with previous work and also confirms the effect of solvate surface layer on the deactivation of carbon surface against parasitic reactions for electrolyte decomposition [7] , [14] . It is noted that the amount of the solvate on pretreated 13 C cathode was not enough to completely eliminate the CO 2 evolution. To study the effect of solvate amount on the elimination of CO 2 evolution, we preloaded the solvate on a glass filter (GF) separator before assembling the cells. 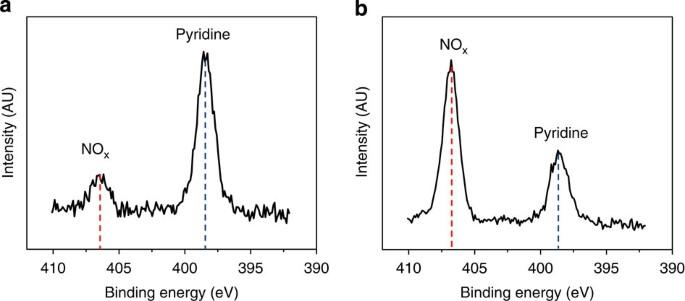Figure 2: XPS on carbon cathode. (a) The N1s XPS result of the carbon cathode after discharge process. The carbon cathode was pretreated with 0.5 M LiNO3-DME to deposit the surface layer. LiTFSI-DME (1 M) was used as the electrolyte. (b) The N1s XPS result of the carbon cathode after discharge process of the cell containing preloaded GF separator. The solvate of LiNO3-DME was preloaded into GF before assembly of the cell. LiTFSI-DME (1 M) was used as the electrolyte. The red and blue dotted lines correspond to the NOxspecies and Pyridinic structure, respectively. Figure 2: XPS on carbon cathode. ( a ) The N1s XPS result of the carbon cathode after discharge process. The carbon cathode was pretreated with 0.5 M LiNO 3 -DME to deposit the surface layer. LiTFSI-DME (1 M) was used as the electrolyte. ( b ) The N1s XPS result of the carbon cathode after discharge process of the cell containing preloaded GF separator. The solvate of LiNO 3 -DME was preloaded into GF before assembly of the cell. LiTFSI-DME (1 M) was used as the electrolyte. The red and blue dotted lines correspond to the NO x species and Pyridinic structure, respectively. Full size image As mentioned above, the solvate of LiNO 3 -DME forms solid phase ionic association. When the solvate was deposited in GF, irregular solid particles were observed at the space between glass fibres ( Supplementary Fig. 8 ). The composition of the solvate was measured using FTIR spectroscopy, which confirms the existence of LiNO 3 and DME molecules ( Supplementary Fig. 9 ). The discharge and charge profiles of the Li–O 2 cell containing the preloaded GF separator with 1 M LiTFSI-DME electrolyte ( Supplementary Fig. 10a ) are very similar to those of the cell containing pristine GF with 0.5 M LiNO 3 -DME electrolyte (shown in Fig. 1b ). The DEMS results show very small amount of CO 2 evolution ( Supplementary Fig. 10b ) at the end of charge process. This suggests that the amount of the solvate on the preloaded GF was enough to significantly suppress the CO 2 evolution. The N1s XPS spectra of the carbon cathode after discharge process evidence the existence of both Pyridinic structure and the surface layer containing NO x species as shown in Fig. 2b . Relatively stronger intensity of NO x peak implies that the formation of surface layer continues during discharge process if the supply of the solvate is not limited. This is in good agreement with the linear increase in R s during discharge cycle as shown in Fig. 1f . The hysteresis in R s at the end of charge cycle in Fig. 1f is attributed to the loss of ionic species by forming Pyridinic structure and the residue of the solvate on carbon surface. This is supported by the XPS result after discharge and charge processes ( Supplementary Figs 11 and 12 ). Mixed electrolytes Generally speaking, solvents with high boiling temperature and/or low vapor pressure are envisioned as ideal when one considers the cycle life and the safety of Li–O 2 cells. As DME has relatively low boiling temperature (85 °C), we tested whether the deactivation of carbon with LiNO 3 -DME solvate is still possible in the presence of high boiling point cosolvent(s). We tested two mixed electrolyte systems: (a) LiNO 3 -DME and LiNO 3 - N , N -dimethylacetamide (DMAc, boiling point (b.p.) of 165 °C) and (b) LiNO 3 -DME and LiNO 3 -tetraethylene glycol dimethyl ether (tetraglyme, b.p. of 275 °C). Strikingly, the results indicated that the deactivation of carbon took place in the mixed electrolytes and the evolution of CO 2 was completely eliminated. 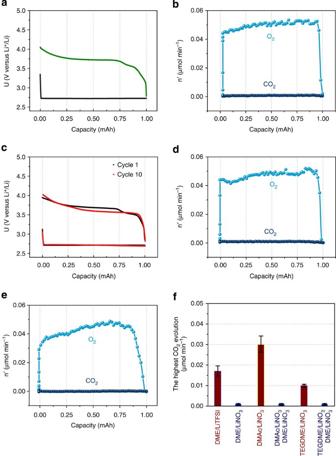Figure 3: Li–O2cells with mixed electrolytes. (a) Galvanostatic discharge/charge profiles and (b)in situDEMS data of the cell containing a mixed electrolyte of 50/50 (wt/wt) 1 M LiNO3-DME and 1 M LiNO3-DMAc. (c) The first (black) and tenth (red) galvanostatic discharge/charge profiles of the cell containing a mixed electrolyte of 50/50 (wt/wt) 1 M LiNO3-DME and 0.5 M LiNO3-tetraglyme. (d)In situDEMS data of the first charge cycle of the cell inc. (e)In situDEMS data of the tenth charge cycle of the cell inc. (f) The peak CO2evolution (μmol min−1) of the cells containing various electrolytes. The results from five cells of each electrolyte were averaged for the statistics. Figure 3a shows the discharge/charge profiles of a Li–O 2 cell containing a 50/50 (wt/wt) mixture of 1 M LiNO 3 -DME and 1 M LiNO 3 -DMAc. The discharge/charge profiles of the mixed electrolyte were similar to those with single electrolyte of 1 M LiNO 3 -DMAc ( Supplementary Fig. 13a ). However, DEMS results showed clear difference in gas evolution. The Li–O 2 cell containing single electrolyte of LiNO 3 -DMAc (as shown in Supplementary Fig. 13b ) evolved fair amount of CO 2 and the experiment with isotope carbon showed the origin of CO 2 was both the electrolyte and the cathode ( Supplementary Fig. 13c,d ). In contrast, the DEMS result in Fig. 3b indicates the complete elimination of CO 2 evolution when mixed electrolyte was used. This evidences that the solvate of LiNO 3 -DME plays its role to deactivate the carbon even in the mixed electrolyte. Figure 3: Li–O 2 cells with mixed electrolytes. ( a ) Galvanostatic discharge/charge profiles and ( b ) in situ DEMS data of the cell containing a mixed electrolyte of 50/50 (wt/wt) 1 M LiNO 3 -DME and 1 M LiNO 3 -DMAc. ( c ) The first (black) and tenth (red) galvanostatic discharge/charge profiles of the cell containing a mixed electrolyte of 50/50 (wt/wt) 1 M LiNO 3 -DME and 0.5 M LiNO 3 -tetraglyme. ( d ) In situ DEMS data of the first charge cycle of the cell in c . ( e ) In situ DEMS data of the tenth charge cycle of the cell in c . ( f ) The peak CO 2 evolution (μmol min −1 ) of the cells containing various electrolytes. The results from five cells of each electrolyte were averaged for the statistics. Full size image The mixing composition of two electrolytes was found to be critical for effective elimination of CO 2 evolution ( Supplementary Fig. 14 ). In fact, for DMAc, the mixed electrolyte with less than 50 wt% of LiNO 3 -DME leads to CO 2 evolution ( Supplementary Fig. 14 ). This implies that to maintain the solvate structure of LiNO 3 -DME in mixed electrolyte solution is essential for the eliminating CO 2 evolution. The nature (such as solubility) and the amount of cosolvent(s), therefore, need to be carefully controlled to avoid the destruction of the solvate. We were also able to operate the CO 2 evolution free Li-O 2 cells using a mixed electrolyte of 50/50 (wt/wt) 0.5 M LiNO 3 -tetraglyme and 1 M LiNO 3 -DME as well ( Fig. 3c–e and Supplementary Fig. 15 ). We summarized the peak CO 2 evolution from mixed electrolytes in Fig. 3f , which suggests that the effect of LiNO 3 -DME solvate on the deactivation of carbon cathode is general. Finally, we confirmed that the elimination of CO 2 evolution is maintained during multiple discharge/charge cycles. Figure 3c,e shows discharge/charge profiles and gas evolutions of the first and tenth cycles, respectively, of the cell containing mixed electrolyte of 50/50 (wt/wt) 1 M LiNO 3 -DME and 0.5 M LiNO 3 -tetraglyme. It is clear that no CO 2 evolution was observed even after tenth cycle of the Li–O 2 cell. The N1s XPS results (not shown here) of the cathode after tenth cycle indicate the formation of Pyridinic structure. It should be noted that the O 2 evolution profile of the tenth charge cycle ( Fig. 3e ) shows reduced amount of O 2 evolution compared with the first cycle. This implies that other parasitic reactions that lower the oxygen efficiency still exist during the cycles, even though the deactivated cathode eliminates the CO 2 evolution. This work demonstrated the elimination of CO 2 evolution from Li–O 2 cells with carbon cathode by mitigating the reactivity of carbon. The surface layer of LiNO 3 -DME solvate on carbon deactivates the carbon surface through the electrochemical nitrogen doping of carbon (during the operation of the Li-O 2 cells), which hinders the parasitic reactions to evolve the CO 2 . It is noted that the nitrogen doping is a result of the reaction between active sites on carbon and the solvate but not a sufficient requirement for the elimination of CO 2 evolution. Ex situ N-doped carbon, for example, may still contain defects that are active to parasitic reactions, and thus leads to CO 2 evolution during the charge process of Li–O 2 cells. The elimination of CO 2 evolution works for mixed electrolytes (as long as the cosolvents do not disturb the solvate structure of LiNO 3 -DME) and for multiple discharge/charge cycles. This work motivates more active research on managing undesired nature of commonly available carbon, which will help to keep the promise of the high specific energy of the Li–O 2 cells. Materials and cathode preparation Battery grade DME, tetraglyme and DMAc solvents were purchased from Novolyte Corp. and dried over 0.4 nm molecular sieves. LiNO 3 and LiTFSI (Novolyte Corp.) salts were dried under high vacuum at 150 °C for 12 h. The water content of solvent and salts is less than 10 p.p.m. measured by Karl Fischer titration. The electrolytes were prepared in an Ar-filled glove box (<0.1 p.p.m. O 2 and H 2 O). The pure Li metal was purchased from FMC and used as received. The GF (GF/C, Whatman) was dried under 150 °C vacuum oven for 24 h. Ketjenblack (KB) carbon (AkzoNobel) or 13 C carbon (Cambridge isotope laboratories, Inc.) was well mixed with a 60 wt% PTFE (Sigma-Aldrich) binder in water solution and subsequently coated on a Toray carbon paper (TGP-H-030). The carbon cathodes were dried under 150 °C vacuum oven for 24 h and transferred to the Ar-filled glove box before the cell fabrication. Fabrication of Li–O 2 Cells Cell fabrication was done in an Ar-filled glove box (<0.1 p.p.m. O 2 and H 2 O). Fabrication of Li–O 2 cells began with placing 11 mm diameter and 250-μm thick Li disc on an anode side current collector. The GF (GF/C, Whatman) was then placed on the Li disc. An electrolyte solution (65 μl) was injected into the GF followed by placing a KB or 13 C carbon cathode and a spacer for head volume of the DEMS cell. Finally, a cathode current collector that has inlet and outlet holes for oxygen gas was placed on top of cathode to complete the cell fabrication. Characterization methods The nanostructure of the KB carbon surface was observed by SEM (Hitachi S-4700) with field emission gun electron microscope. For transferring the KB cathode samples to SEM chamber, the Li–O 2 cells were disassembled in an Ar-filled glove box after discharge or discharge-charge process. The KB cathodes were stored in an Ar-filled plastic carrier. The sample was transferred to the SEM anti-chamber and immediately evacuated the chamber (less than 5 s). The surface of cathodes was investigated by XPS (An Omicron, ESCA probe spectrometer) using monochromatic Al K-alpha radiation (1,486.6 eV) with 200 μm spot size throughout and charge neutralization under vacuum of ~10 −10 Torr. The XPS samples were prepared in an Ar-filled glove box after discharge or discharge-charge process and transferred with an Ar-filled carrier. Surface atomic concentration percent ( C i ) was estimated using the equation C i =I i /σ i /Σ I n /σ n , where I is the peak area and σ the energy corrected photoionization cross-section of the i th element. This calculation assumed uniform composition with depth. Electrochemical measurements were performed using a BioLogic VMP3 Multichannel Workstation. The details of DEMS system were described elsewhere [12] . The X-ray diffraction analysis of the Li 2 O 2 crystals was performed using a Bruker D8 DISCOVER GADDS Series. How to cite this article: Kang, S. J. et al. Deactivation of carbon electrode for elimination of carbon dioxide evolution from rechargeable lithium–oxygen cells. Nat. Commun. 5:3937 doi: 10.1038/ncomms4937 (2014).